CBR antimicrobials alter coupling between the bridge helix and the β subunit in RNA polymerase Bacterial RNA polymerase (RNAP) is a validated target for antibacterial drugs. CBR703 series antimicrobials allosterically inhibit transcription by binding to a conserved α helix (β′ bridge helix, BH) that interconnects the two largest RNAP subunits. Here we show that disruption of the BH-β subunit contacts by amino-acid substitutions invariably results in accelerated catalysis, slowed-down forward translocation and insensitivity to regulatory pauses. CBR703 partially reverses these effects in CBR-resistant RNAPs while inhibiting catalysis and promoting pausing in CBR-sensitive RNAPs. The differential response of variant RNAPs to CBR703 suggests that the inhibitor binds in a cavity walled by the BH, the β′ F-loop and the β fork loop. Collectively, our data are consistent with a model in which the β subunit fine tunes RNAP elongation activities by altering the BH conformation, whereas CBRs deregulate transcription by increasing coupling between the BH and the β subunit. RNA polymerase (RNAP) mediates synthesis of an RNA copy of the template DNA—the first and often decisive step in gene expression. All RNAPs transcribing cellular genomes are multisubunit enzymes that share homologous catalytic cores [1] , [2] . Bacterial RNAP, a five-subunit complex ααββ′ω, is the simplest model system for studies of fundamental mechanistic properties of all multisubunit RNAPs and a validated target for antibacterial drugs [3] . The cycle of nucleotide incorporation by RNAP is governed by alternate closure and opening of the active site by a β′ subunit mobile domain called trigger loop (TL): catalysis of phospho-diester bond formation involves an obligatory closure [4] , [5] , whereas translocation along the DNA requires opening of the active site [6] . RNAP also reversibly isomerizes into an off-pathway state that is inhibitory for nucleotide addition. The off-pathway state, aka an elemental pause [7] , is the precursor to all regulatory events during transcription elongation, such as longer-lived pauses and termination [8] , [9] , [10] . Long-lived pauses in turn function to synchronize transcription and translation in prokaryotes [11] , [12] and to recruit regulatory proteins to transcribing RNAP in all domains of life [13] , [14] , [15] . The structural rearrangements accompanying catalysis are relatively well understood. The TL folding into a closed conformation is dependent on the formation of a triple-helical bundle with the β′ subunit bridge helix (BH), a long metastable α helix that spans the active site cleft and moulds into a groove in the β subunit [4] ( Fig. 1a ). The stability of folded TL is also modulated by its interaction with the β′ F-loop, an amino-terminal extension of BH [16] . The structural rearrangements associated with isomerization into the elemental pause remain elusive owing to the transient nature of the state. It has been suggested that this isomerization involves fraying of the RNA 3′-end in the active site, kinking of the BH, opening of the β′ clamp domain and changes in the template DNA conformation in the vicinity of the active site [8] , [17] , [18] , [19] , [20] . 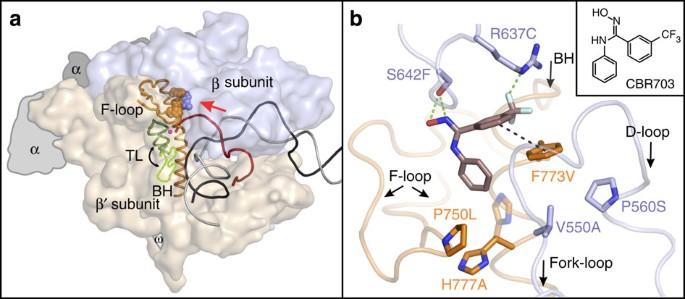Figure 1: Binding site of CBR series inhibitors at the BH-β subunit interface. (a) An overview of the bacterial TEC. β (light blue) and β′ (wheat) are depicted as semi-transparent surfaces, α and ω (largely obstructed by β′) subunits are depicted as flat grey outlines. BH (orange), F-loop (orange), TL (green—closed conformation, dashed light green—open conformation), RNA (red), template (black) and non-template (grey) DNA strands are depicted as cartoons. Amino-acid residues altered in this study are depicted as spheres. A red arrow indicates the direction of the view inb. (b) CBR703 (sticks with brown carbons and inset) docked at the BH-β subunit interface ofE. coliRNAP (PDB 4IGC)37. The native amino-acid residues replaced by CBR703-resistant and -sensitive (βP560S and β′H777A) substitutions are depicted as sticks. Cartoons and side chain’s carbons of β and β′ are coloured pastel blue and orange, respectively. The outwards37,50,51(opaque) and inwards52(semi-transparent) facing conformers ofE. coliβ′His777 are shown. Green and black-dashed lines depict polar and π-stacking interactions, respectively. Figure was prepared using PyMOL Molecular Graphics System, Version 1.6.0.0; Schrödinger, LLC. The sources of atomic coordinates are listed inSupplementary Table 3. Figure 1: Binding site of CBR series inhibitors at the BH-β subunit interface. ( a ) An overview of the bacterial TEC. β (light blue) and β′ (wheat) are depicted as semi-transparent surfaces, α and ω (largely obstructed by β′) subunits are depicted as flat grey outlines. BH (orange), F-loop (orange), TL (green—closed conformation, dashed light green—open conformation), RNA (red), template (black) and non-template (grey) DNA strands are depicted as cartoons. Amino-acid residues altered in this study are depicted as spheres. A red arrow indicates the direction of the view in b . ( b ) CBR703 (sticks with brown carbons and inset) docked at the BH-β subunit interface of E. coli RNAP (PDB 4IGC) [37] . The native amino-acid residues replaced by CBR703-resistant and -sensitive (βP560S and β′H777A) substitutions are depicted as sticks. Cartoons and side chain’s carbons of β and β′ are coloured pastel blue and orange, respectively. The outwards [37] , [50] , [51] (opaque) and inwards [52] (semi-transparent) facing conformers of E. coli β′His777 are shown. Green and black-dashed lines depict polar and π-stacking interactions, respectively. Figure was prepared using PyMOL Molecular Graphics System, Version 1.6.0.0; Schrödinger, LLC. The sources of atomic coordinates are listed in Supplementary Table 3 . 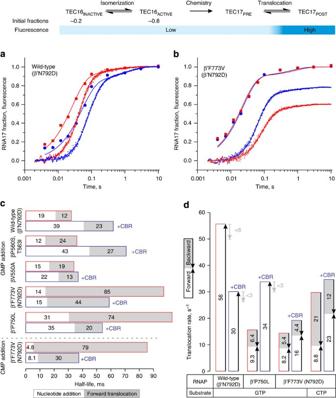Figure 3: Effects of CBR703 and substitutions at the BH-β subunit interface on nucleotide addition and translocation rates. Top schematic describes the experimental set-up. CBR703 is present at 100 μM where indicated (blue outline). Best fit curves and bar graphs were drawn using parameters described inSupplementary Table 5. (a,b) Time courses of GMP addition (discrete time points) and translocation (continuous trace) by wild-type (a) and β′F773V (b) RNAPs. Nucleotide addition and translocation assays were performed in duplicate; translocation curves are averages from six to nine time traces. (c) Half-lives of nucleotide addition cycles calculated as sums of nucleotide addition (white fill) and forward translocation (grey fill) half-lives. (d) The apparent translocation rates of wild-type (β′N792D), β′P750L and β′F773V, β′N792D RNAPs depicted as sums of forward (white fill) and backward (grey fill) translocation rates. The representation reflects the relationship between the above three rates defined by formal kinetic rules for a reversible reaction. For wild-type RNAP and β′P750L (in the presence of CBR703), the backward rates are constrained to zero during the fit but may potentially constitute up to 10% of forward rate (grey arrows) assuming 10% uncertainty in determination of fluorescent levels of extended TECs. Full size image RNAP active site structure evolved to achieve optimal balance between catalytic efficiency, processivity and amenability to regulation [21] . First, the stability of folded TL is tuned up to permit both efficient catalysis and rapid translocation that require folding and unfolding of TL, respectively. Second, the propensity to isomerize into the elemental paused state is tuned up to permit both efficient RNA chain elongation and the proper response to regulatory signals. In this work, we present evidence that conformational coupling between the β subunit and BH plays an important role during elongation by RNAP. We also report plausible structural models of CBR703 ( N -hydroxy- N ′-phenyl-3-trifluoromethyl-benzamidine) series inhibitors [22] , [23] bound in an occluded pocket at the BH-β subunit interface and elucidate mechanistic details of their antibacterial action. RNAPs with amino-acid substitutions at BH-β interface To gain insights into the mechanism of action of CBR-type antibiotics, we performed the detailed analysis of elongation activities of five RNAPs with substitutions at the BH-β subunit interface, the anticipated binding site of CBRs ( Fig. 1b ). The BH β′F773V and F-loop β′P750L were first identified in a genetic screen for alleles resistant to CBR-type inhibitors [22] . β′F773V RNAP was later characterized as pause and terminator resistant [24] and has been suggested to have altered translocation and fidelity [25] . The D-loop βP560S,T563I (RpoB5101) RNAP was identified in an in vivo screen as an enzyme with decreased termination [26] . The Fork loop βV550A RNAP was designed to probe interactions of β′F773 with the β Fork loop. The BH β′H777A RNAP was reported to have relatively unaltered in vitro activity and mild in vivo growth defects in a study by Jovanovic et al . [27] Here we reevaluated β′H777A properties to probe the clash between CBR703 and one of the β′H777 conformers revealed by docking experiments (see below). Most of experiments in this study were performed with wild type and β′F773V RNAPs that also contained a BH β′N792D substitution. The β′N792D substitution increased Escherichia coli RNAP sensitivity to streptolydigin (STL) [28] but did not detectably affect the nucleotide addition and translocation rates as well as translocation bias (this work), enabling us to use low concentrations of STL, which do not interfere with fluorescence measurements, to bias RNAP forward in translocation studies. We assembled variant RNAP transcription elongation complexes (TECs) on chemically synthesized nucleic-acid scaffolds containing fluorescent 6-methyl-isoxanthopterin (6-MI) base in the template strand and used direct time-resolved translocation [6] and nucleotide-addition [29] , [30] assays to study the effects of substitutions on RNAP translocation equilibrium, translocation rates, catalytic activity and response to CBR703. We also compared effects of these substitutions on RNAP response to a regulatory pause site in the presence and absence of CBR703. β′F773V and β′P750L backward bias translocation equilibrium All five variant RNAPs translocated forward following the incorporation of the cognate GMP, as judged by increase in 6-MI fluorescence. To assess the completeness of translocation, we compared fluorescence intensities of TECs extended by rNMP and 2′dNMP. The 2′dNMP-extended TECs are anticipated to display higher level of fluorescence than the rNMP-extended TECs unless the latter are fully post-translocated because 2′ OH group is essential for stabilizing the pre-translocated state [6] . The 2′dNMP-extended β′F773V and β′P750L TECs displayed brighter fluorescence than the rNMP-extended TECs ( Fig. 2a and Supplementary Fig. 1 ). In contrast, the fluorescence levels of GMP- and 2′dGMP-extended TECs formed by other RNAPs were the same. Forward-biasing 3′dNMP- and rNMP-extended β′F773V and β′P750L TECs with the next incoming substrate NTPs and their non-hydrolyzable analogues, respectively, reported fluorescence levels similar to those of the 2′dNMP-extended TECs ( Fig. 2a and Supplementary Fig. 1 ). We concluded that the 2′dNMP-extended β′F773V and β′P750L TECs are nearly 100% post-translocated, whereas AMP- or GMP-extended TECs contain ~40% and CMP- or UMP-extended TECs contain ~70% of pre-translocated state. 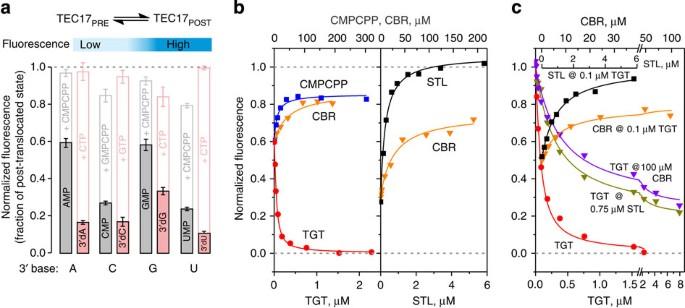Overall, the above experiments revealed that β′F773V and β′P750L RNAPs displayed a measurable fraction of pre-translocated states, whereas other RNAPs in our set were nearly 100% post-translocated. Figure 2: Effects of CBR703 and substitutions at the BH-β subunit interface on translocation equilibrium. Top schematic describes the experimental set-up. Best fit curves were simulated using parameters described inSupplementary Table 4. Fluorescence data were averaged over two to three experiments. (a) β′F773V TECs display measurable fractions of the pre-translocated state. Fluorescence of rNMP (grey fill) and 3′dNMP (pink fill)-extended TECs normalized to the level of 2′dNMP-extended TECs. White bars depict the effects of the next substrate NTP (pink outline) or its non-hydrolyzable analogue (grey outline). Error bars are s.d. (b) CBR703 and STL forward-biased β′F773V RNAP sensitized to STL by the β′N792D substitution. Left panel: GMP-extended TEC. Right panel: CMP-extended TEC. TGT (red) and STL (black) quantitatively move the TECs into pre- and post-translocated states, respectively. CBR703 (orange) and cytidine-5′-[(α,β)-methyleno]triphosphate (CMPCPP; blue) measurably forward bias the TECs. (c) STL and CBR703 offset TGT effects on wild-type RNAP sensitized to STL by β′N792D substitution. TGT (red) quantitatively converts post-translocated GMP-extended TEC into pre-translocated TEC. TGT is less potent in backward-biasing RNAP in the presence of 0.75 μM STL (olive) and 100 μM CBR703 (purple). STL (black) and CBR703 (orange) forward bias RNAP in the presence of 0.1 μM TGT. Figure 2: Effects of CBR703 and substitutions at the BH-β subunit interface on translocation equilibrium. Top schematic describes the experimental set-up. 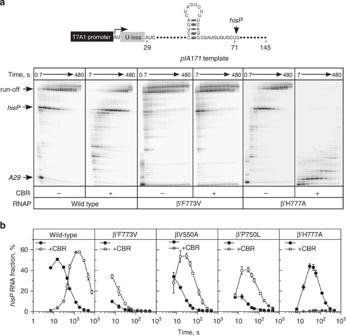Figure 4: Effects of CBR703 and substitutions at the BH-β subunit interface on pausing at the regulatory pause site. (a) Transcript elongation on pIA171 template by wild-type, β′F773V and β′H777A RNAPs in the absence (left panels) or in the presence (right panels) of 100 μM CBR703. (b) Quantification of the fraction of RNA at thehisP(transcript position U71) from the data shown inaandSupplementary Fig. 3. Fraction refers to the ratio of the paused RNA to the sum of all products resulting from elongation of TEC halted at A29. Error bars are s.d. of three independent experiments. Best fit curves were simulated using parameters described in Supplementary Table 4 . Fluorescence data were averaged over two to three experiments. ( a ) β′F773V TECs display measurable fractions of the pre-translocated state. Fluorescence of rNMP (grey fill) and 3′dNMP (pink fill)-extended TECs normalized to the level of 2′dNMP-extended TECs. White bars depict the effects of the next substrate NTP (pink outline) or its non-hydrolyzable analogue (grey outline). Error bars are s.d. ( b ) CBR703 and STL forward-biased β′F773V RNAP sensitized to STL by the β′N792D substitution. Left panel: GMP-extended TEC. Right panel: CMP-extended TEC. TGT (red) and STL (black) quantitatively move the TECs into pre- and post-translocated states, respectively. CBR703 (orange) and cytidine-5′-[(α,β)-methyleno]triphosphate (CMPCPP; blue) measurably forward bias the TECs. ( c ) STL and CBR703 offset TGT effects on wild-type RNAP sensitized to STL by β′N792D substitution. TGT (red) quantitatively converts post-translocated GMP-extended TEC into pre-translocated TEC. TGT is less potent in backward-biasing RNAP in the presence of 0.75 μM STL (olive) and 100 μM CBR703 (purple). STL (black) and CBR703 (orange) forward bias RNAP in the presence of 0.1 μM TGT. Full size image β′F773V RNAP translocation is controlled by TL opening We employed two antibiotics with established modes of action, tagetitoxin (TGT) and STL, to demonstrate that translocation of β′F773V TEC is controlled by opening and closure of the active site by the TL. TGT is a high-affinity pyrophosphate analogue that backward biases RNAP by stabilizing the closed active site [6] , [31] . Indeed, addition of saturating amounts of TGT to rNMP-extended TECs reduced their fluorescence to the level of non-extended TECs, which corresponds to the pre-translocated state ( Fig. 3 ). STL binds to the inner face of the BH and stabilizes the open active site conformation, favouring the post-translocated state [28] , [32] . Indeed, addition of saturating amounts of STL to rNMP-extended TECs increased their fluorescence to the level of 2′dNMP-extended TECs, which correspond to the post-translocated state ( Fig. 2b ). CBR703 also forward biased β′F773V TECs in a concentration-dependent manner, although it was less potent than STL and failed to quantitatively move the TECs into the post-translocated state ( Fig. 2b ). Both STL and CBR703 forward biased wild-type RNAP, as evident from their ability to offset the effect of TGT on translocation equilibrium ( Fig. 2c ). The response of β′F773V RNAP to STL suggests that the shift of translocation equilibrium towards the pre-translocated state in this RNAP originates, at least in part, from an increased stability of the folded TL. The ability of CBR703 to forward bias β′F773V and wild-type RNAPs suggests that the inhibitor destabilizes the folded TL. Figure 3: Effects of CBR703 and substitutions at the BH-β subunit interface on nucleotide addition and translocation rates. Top schematic describes the experimental set-up. CBR703 is present at 100 μM where indicated (blue outline). 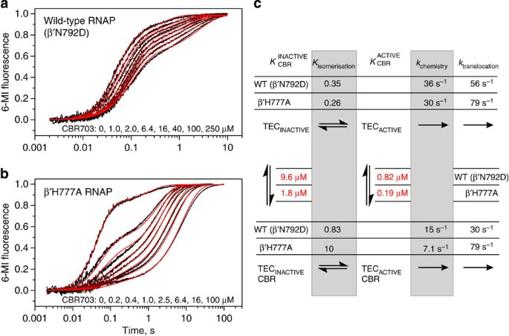Figure 5: CBR703 slows down catalysis and promotes isomerization into the inactive state. Wild-type (a) and β′H777A (b) TEC16s are preincubated with different concentrations of CBR703, rapidly mixed with GTP and formation of post-translocated TEC17s is monitored by continuous recording of 6-MI fluorescence (black traces). Best fit curves (red) were simulated using parameters described incandSupplementary Methods. The experiments were performed in duplicate, fluorescence curves are averages from three to seven time traces. (c) Kinetic scheme describing the effects of CBR703 on completion of GMP addition cycle inaandb. Grey boxes and red font accentuate parameters affected by CBR703 and β′H777A substitution, respectively. Best fit curves and bar graphs were drawn using parameters described in Supplementary Table 5 . ( a , b ) Time courses of GMP addition (discrete time points) and translocation (continuous trace) by wild-type ( a ) and β′F773V ( b ) RNAPs. Nucleotide addition and translocation assays were performed in duplicate; translocation curves are averages from six to nine time traces. ( c ) Half-lives of nucleotide addition cycles calculated as sums of nucleotide addition (white fill) and forward translocation (grey fill) half-lives. ( d ) The apparent translocation rates of wild-type (β′N792D), β′P750L and β′F773V, β′N792D RNAPs depicted as sums of forward (white fill) and backward (grey fill) translocation rates. The representation reflects the relationship between the above three rates defined by formal kinetic rules for a reversible reaction. For wild-type RNAP and β′P750L (in the presence of CBR703), the backward rates are constrained to zero during the fit but may potentially constitute up to 10% of forward rate (grey arrows) assuming 10% uncertainty in determination of fluorescent levels of extended TECs. Full size image Altered RNAPs have decreased forward translocation rate We performed parallel time-resolved measurements of nucleotide addition and translocation for GMP (and CMP in case of β′F773V RNAP) addition reactions. The forward and backward translocation rates were inferred from a delay between nucleotide addition and translocation curves using a reversible translocation model, as described in Supplementary Methods . These analyses revealed that RpoB5101 and βV550A substitutions reduced the forward translocation rate to 30–40 s −1 (from 60 s −1 in wild-type RNAP), whereas β′F773V and β′P750L substitutions reduced the rate to 9 s −1 ( Fig. 3 and Supplementary Fig. 2 ). The backward translocation rate was estimated at 6 s −1 for GMP-extended β′F773V and β′P750L TECs and at 20 s −1 for CMP-extended β′F773V TEC ( Fig. 3d ), but did not measurably contribute to the kinetics of fluorescence change in other RNAPs and was fixed to zero during analyses. Whereas the 6s −1 rate could be potentially masked by 60 s −1 forward translocation rate in wild-type RNAP (assuming 10% uncertainly in determination of equilibrium levels of fluorescence), the 20s −1 value strongly suggests that β′F773V substitution increases backward translocation rate. The shift of translocation equilibrium towards the pre-translocated state in β′F773V RNAP thus originates from both the decrease in forward and increase in backward translocation rates. The decrease in BH mobility or bendability [25] alone is not sufficient to explain such observations, whereas stabilization of the folded TL, in part as a consequence of less bendable BH, satisfactory explains the observed effects. Altered RNAPs are differentially sensitive to CBR703 We investigated the effect of CBR703 on nucleotide addition and translocation rates of variant RNAPs in the single nucleotide addition assay. Preincubation of TECs with 100 μM CBR703 lengthened nucleotide addition cycle twofold in the wild-type and RpoB5101 RNAPs, had little effect on βV550A and facilitated the completion of the cycle by β′P750L and β′F773V RNAPs twofold ( Fig. 3c ). β′H777A RNAP was inhibited nearly 250-fold and is discussed in a separate section (see below). At the level of individual steps, nucleotide addition was unaffected or inhibited, whereas forward translocation was marginally inhibited in wild-type RNAP, unaffected in RpoB5101 and stimulated in βV550A, β′P750L and β′F773V RNAPs ( Fig. 3c ). CBR703 also reduced backward translocation rate of β′P750L TEC below the detection threshold and marginally slowed-down backward translocation of β′F773V TECs ( Fig. 3d ). The effect of CBR703 on translocation rates of β′P750L and β′F773V RNAPs is consistent with its forward-biasing effect in the equilibrium assay ( Fig. 2b ) and reinforces the hypothesis that inhibitor promotes the TL unfolding. Consistently, with the results of single nucleotide addition assays, CBR703 permitted rapid processive transcription through the long template by β′F773V, β′P750L and βV550A RNAPs ( Fig. 4 and Supplementary Fig. 3 ). In contrast, transcription by wild-type RNAP was significantly impeded by multiple pauses. Figure 4: Effects of CBR703 and substitutions at the BH-β subunit interface on pausing at the regulatory pause site. ( a ) Transcript elongation on pIA171 template by wild-type, β′F773V and β′H777A RNAPs in the absence (left panels) or in the presence (right panels) of 100 μM CBR703. ( b ) Quantification of the fraction of RNA at the hisP (transcript position U71) from the data shown in a and Supplementary Fig. 3 . Fraction refers to the ratio of the paused RNA to the sum of all products resulting from elongation of TEC halted at A29. Error bars are s.d. of three independent experiments. Full size image Altered RNAPs have reduced sensitivity to regulatory pause β′F773V and RpoB5101 RNAPs are among the least pause responsive E. coli RNAPs hitherto characterized [24] . To find out whether pause insensitivity is a general property of RNAPs with substitutions at the BH-β subunit interface, we evaluated their response to the hairpin-stabilized hisP pause element using a standard single-round in vitro transcription assay [33] . We used the pIA171 linear transcription template on which the hisP was positioned downstream from a strong T7A1 promoter ( Fig. 4 ). On this template, radiolabelled transcription complexes can be halted at position A29 when transcription is initiated in the absence of UTP, with ApU dinucleotide, ATP, GTP and α–[ 32 P]CTP. The halted A29 complexes can then be chased on addition of all four NTP substrates. We found that, similar to β′F773V and RpoB5101 RNAPs characterized earlier [24] , β′P750L and βV550A RNAPs were relatively resistant to the hisP pause ( Fig. 4 and Supplementary Fig. 3 ), suggesting that weakening BH-β subunit contacts universally leads to insensitivity to regulatory pauses. Strikingly, the sensitivity of β′F773V, β′P750L and βV550A RNAPs to hisP pause was partially restored in the presence of CBR703. The latter result suggests that CBR703 promotes formation of native intermediates in the pausing pathway. In silico docking of CBRs at the BH-β interface It has been anticipated for some time that CBR-type compounds bind at the BH-β subunit interface of E. coli RNAP near β'F773 based on extensive set of in vivo selected CBR703- and CBR9379-resistant mutations [22] . Here we used AutoDock Vina [34] and GOLD [35] , [36] programs, which rely on different algorithms and scoring functions, to identify the binding sites for CBR703, CBR9379 and CBR9393 in E. coli RNAP holoenzyme crystal structure (PDB 4IGC) [37] . Both Vina and GOLD failed to identify a common binding mode for the three inhibitors to rigid RNAP but robustly recovered overlapping binding sites for CBR9379 and CBR9393 when β′Leu770 and β′Phe773 side chains were set flexible ( Supplementary Fig. 4 ). Moreover, Vina independently recovered the same binding mode for CBR703 ( Fig. 1b ), a relatively symmetric substructure of CBR9379. In the resulting models, the structural moieties common for the three CBRs are positioned in a spacious cavity walled by the BH, Fork loop and F-loop and interact with key residues implicated in resistance to CBRs ( Fig. 1b and Supplementary Fig. 4 ) Trifluoromethyl group forms hydrogen bond with βArg637 and interacts with aromatic π-system of β′Phe773. Trifluoromethylated benzene ring stacks with β′Phe773 in an offset parallel configuration, whereas the second benzene ring contacts β′Pro750, β′Ile774 and βVal550. The N -hydroxyamidine moieties interconnecting benzene rings in CBR703 and CBR9379 interact with hydroxyl group and main chain carbonyl of βSer642. Bulky substituents in position 4 (in CBR9393) and 5 (in CBR9379) of trifluoromethylated ring extend into β lobe, form multiple van der Waals interactions with RNAP side chains and hydrogen bond with βGlu611 (in CBR9393–RNAP complex) and βPro552 main chain carbonyl (in CBR9379–RNAP complex) accounting for higher potency of the larger CBRs ( Supplementary Fig. 4 ). The atomic coordinates of CBR703, CBR9379 and CBR9393–RNAP complexes are provided as Supplementary Data 1–3 , respectively. We noted that in Thermus thermophilus RNAP structures, the orientation of the BH β′His1075 side chain is different from that of the homologous β′His777 in the crystal structure of E. coli RNAP holoenzyme that we used for docking experiments. The β'His1075 side chain extends into the CBR703-binding cavity and clashes with the unsubstituted aromatic ring of CBR703 ( Fig. 1b ). This observation suggests that the E. coli β'His777 side chain may alternate between the inwards and outwards facing conformations, interfering with CBRs binding in the former state. In support of the docking model, the β'H777A substitution increased E. coli RNAP affinity for CBR703 fivefold ( Fig. 5 ). Figure 5: CBR703 slows down catalysis and promotes isomerization into the inactive state. Wild-type ( a ) and β′H777A ( b ) TEC16s are preincubated with different concentrations of CBR703, rapidly mixed with GTP and formation of post-translocated TEC17s is monitored by continuous recording of 6-MI fluorescence (black traces). Best fit curves (red) were simulated using parameters described in c and Supplementary Methods . The experiments were performed in duplicate, fluorescence curves are averages from three to seven time traces. ( c ) Kinetic scheme describing the effects of CBR703 on completion of GMP addition cycle in a and b . Grey boxes and red font accentuate parameters affected by CBR703 and β′H777A substitution, respectively. Full size image CBR703 promotes TEC isomerization into an inactive state All assembled TECs that we characterized to date contain 5–25% of a slow reacting TEC (1-2 s −1 ) [6] . The slow fraction originates at or before the nucleotide addition step, but is only well resolved in translocation traces because of dense temporal sampling. We noted that CBR703 increased the fraction of slow TEC in CBR-sensitive (wild type and RpoB5101) but not CBR-resistant (βV550A and β'F773V) RNAPs ( Fig. 3 and Supplementary Fig. 2 ). The increase in fraction of slow TEC is particularly apparent in a set of translocation time curves of the wild-type RNAP recorded at increasing concentration of CBR703 ( Fig. 5a ) and becomes explicit when the CBR-hypersensitive β′H777A RNAP is used ( Fig. 5b ). We found that the simplest kinetic model consistent with the wild-type and β′H777A RNAPs data postulates that the slow TEC is an inactive TEC in slow equilibrium with an active TEC ( Fig. 5c ). Note that such definition of a slow TEC matches the definition of a paused TEC. The isomerization rate constants were also in the order of those estimated for the elemental pause in single molecule experiments [9] , [38] . The model predicts that CBR has a dual effect on transcription: it slows down nucleotide addition twofold and promotes isomerization of active TECs into inactive TECs. A stronger effect of CBR703 on β′H777A RNAP originates from changes in two distinct equilibriums: first, the substitution increases CBR703-binding affinity fivefold; second, CBR703 increases bias towards the inactive state 38-fold in β′H777A RNAP ( K iso =0.26, K iso CBR =10) but has only 2.5-fold effect in the wild-type RNAP ( K iso =0.35, K iso CBR =0.83). The capacity of CBR703 to promote TEC isomerization into an inactive state inferred from single nucleotide addition experiments in Fig. 5 is entirely consistent with the CBR703 effects on transcription through the long template in Fig. 4 and Supplementary Fig. 3 , where CBR703 gradually halts β′H777A RNAP at multiple sites and restores pause sensitivity of CBR-resistant RNAPs. Collectively, our data are consistent with the model where disruption of the BH-β subunit contacts relaxes RNAP into a ground state characterized by the predominantly closed active site, fast and error-prone catalysis, slow translocation and insensitivity to regulatory pauses. β′F773V RNAP is a quintessential example of such RNAP. In contrast, in the wild-type RNAP, motions of the β subunit modulate on-pathway elongation and isomerization into off-pathway states ( Fig. 6 ). Specifically, conformational coupling between the BH and β subunit destabilizes BH–TL interactions in a controllable manner, thereby fine tuning translocation and catalysis. Perhaps independently, the β subunit–BH interactions also control the equilibrium between the active and paused states of the TEC via the BH anchor and switch 1 regions [19] , [20] , [39] , [40] . 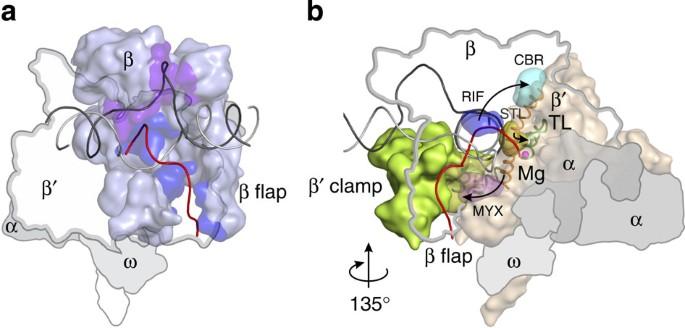Figure 6: Antibiotic-binding sites outline an allosteric path mediating regulation of transcription elongation. (a) The β subunit (light blue) interacts with nucleic-acid determinants implicated in regulation of transcription elongation53,54,55,56: the nascent RNA57(red, blue β surface) and unpaired non-template DNA52,58(black, purple β surface). β′ subunit is depicted as a contour, and α and ω subunits as grey outlines. (b) Allosteric effects (black arrows) travel through rifampicin (RIF, sterically59and allosterically60inhibits transcription initiation) -binding site (blue surface, amino-acid substitutions alter RNAP pausing propensities26) in the β subunit. CBR (inhibits transcription elongation by promoting pausing)-binding site (cyan surface, amino-acid substitutions lead to pausing defects) outlines the interface where allosteric effects are transferred to the BH (orange cartoon). STL (inhibits transcription elongation by restricting TL and BH conformations28,32) -binding site (yellow surface) marks the region where conformational changes in BH modulate the stability of the folded TL (green cartoon). Myxopyronin (restricts mobility of the β′ clamp61,62,63and alters position of template DNA strand64) binds to the flexible region (pink surface, switch 1 as green cartoon on the background) that controls movement of β′ clamp (green surface) and conformation of the template DNA strand (grey cartoon). β subunit is depicted as a contour, and α and ω subunits as grey outlines. The figure was prepared using PyMOL Molecular Graphics System, Version 1.6.0.0; Schrödinger, LLC. The sources of atomic coordinates are listed inSupplementary Table 3. Figure 6: Antibiotic-binding sites outline an allosteric path mediating regulation of transcription elongation. ( a ) The β subunit (light blue) interacts with nucleic-acid determinants implicated in regulation of transcription elongation [53] , [54] , [55] , [56] : the nascent RNA [57] (red, blue β surface) and unpaired non-template DNA [52] , [58] (black, purple β surface). β′ subunit is depicted as a contour, and α and ω subunits as grey outlines. ( b ) Allosteric effects (black arrows) travel through rifampicin (RIF, sterically [59] and allosterically [60] inhibits transcription initiation) -binding site (blue surface, amino-acid substitutions alter RNAP pausing propensities [26] ) in the β subunit. CBR (inhibits transcription elongation by promoting pausing)-binding site (cyan surface, amino-acid substitutions lead to pausing defects) outlines the interface where allosteric effects are transferred to the BH (orange cartoon). STL (inhibits transcription elongation by restricting TL and BH conformations [28] , [32] ) -binding site (yellow surface) marks the region where conformational changes in BH modulate the stability of the folded TL (green cartoon). Myxopyronin (restricts mobility of the β′ clamp [61] , [62] , [63] and alters position of template DNA strand [64] ) binds to the flexible region (pink surface, switch 1 as green cartoon on the background) that controls movement of β′ clamp (green surface) and conformation of the template DNA strand (grey cartoon). β subunit is depicted as a contour, and α and ω subunits as grey outlines. The figure was prepared using PyMOL Molecular Graphics System, Version 1.6.0.0; Schrödinger, LLC. The sources of atomic coordinates are listed in Supplementary Table 3 . Full size image From a structural perspective, decoupling from the β subunit enables the BH to adopt its native helical conformation and to form multiple interactions with the folded TL, thereby promoting the active site closure. The lack of β-induced distortions in the BH structure also diminishes transitions associated with pausing: isomerization of template DNA strand and opening of the clamp domain, which have been structurally linked to the distorted BH [20] , [41] . In contrast, binding of CBR inhibitors fills the void at the BH-β subunit interface and strengthens β subunit interactions with the BH. As a result, the BH–TL interactions are weakened, the folded TL is destabilized and catalysis is slowed down. The β subunit also induces larger distortions in the BH conformation, increasing RNAP propensity to isomerize into inactive state(s) that kinetically resembles the natural intermediates of the pausing pathway. The latter effect may play the major role in the antibacterial action of CBR inhibitors. Whereas the threefold decrease in elongation rate slows down bacterial growth, a small increase in propensity to isomerize into the inactive state at each sequence position increases the frequency of long-lived pause and arrest events, ultimately leading to premature cessation of transcription that is detrimental for cell viability. Similarly, we hypothesize that deregulated transcription, rather than the slow forward translocation rate, makes β′F773V and β′P750L RNAPs inviable in the absence of CBRs [22] . Binding of CBR inhibitors restores the coupling between the BH and β subunit in these RNAPs, thereby restoring transcriptional regulation and supporting viability of the mutant strains. Proteins and reagents DNA and RNA oligonucleotides were purchased from IBA Biotech (Göttingen, Germany) and Fidelity Systems (Gaithersburg, MD, USA). TGT was from Epicentre (Madison, WI, USA), CBR703 from Maybridge (Tintagel, UK) and STL from Sourcon-Padena (Tübingen, Germany). Cytidine-5′-[(α,β)-methyleno]triphosphate and guanine-5′-[(α,β)-methyleno]triphosphate were from Jena Bioscience (Jena, Germany). RNAPs and yeast inorganic pyrophosphatase were expressed and purified as described previously [42] , [43] . Plasmids are listed in Supplementary Table 1 . Template strand oligonucleotides and RNA primers are listed in Supplementary Table 2 . Schematics of all nucleic-acid scaffolds used in this study are shown in Supplementary Fig. 5 . TEC assembly TECs (1 μM) were assembled by a procedure developed by Komissarova et al . [44] An RNA primer labelled with Atto680 fluorescent dye at the 5′-end was annealed to template DNA, and incubated with 1.5 μM RNAP for 10 min at 25 °C in TB10D buffer (10 mM MgCl 2 , 40 mM HEPES-KOH pH 7.5, 80 mM KCl, 5% glycerol, 2.5% dimethylsulphoxide, 0.1 mM EDTA and 0.1 mM DTT) and with 2 μM of the non-template DNA for 20 min at 25 °C. For TECs used in nucleotide addition measurements, RNA was the limiting component at 1 μM and the template strand was used at 1.4 μM, whereas for TECs used in translocation, the template strand was limiting at 1 μM and RNA was added at 1.4 μM. Nucleotide addition measurements To determine the incorporation efficiency of NTP, 2′ and 3′dNTP substrates, 1 μM TEC in 20 μl of TB10D buffer was incubated for 10 min with 5 μM substrates at 25 °C and quenched by adding 80 μl of loading buffer (94% formamide, 13 mM Li 4 -EDTA and 0.2% Orange G). Time-resolved measurements were performed in an RQF 3 quench-flow instrument (KinTek Corporation, Austin, TX, USA). The reaction was initiated by rapid mixing of 14 μl of 0.4 μM TEC with 14 μl of 400 μM NTP. Both TEC and NTP solutions were prepared in TB10D buffer and, where indicated, supplemented with 100 μM CBR703. The reaction was allowed to proceed for 0.004–10 s at 25 °C, quenched with 86 μl of 0.5 M HCl and immediately neutralized by adding 171 μl of loading buffer (290 mM Tris base, 13 mM EDTA, 0.2% Orange G, 94% formamide). RNAs were separated on 16% denaturing polyacrylamide gels and visualized with Odyssey Infrared Imager (Li-Cor Biosciences, Lincoln, NE, USA); band intensities were quantified using ImageJ software [45] . Translocation measurements RNAP translocation was assayed by monitoring changes in fluorescence of 6-MI base incorporated into template DNA [6] . Equilibrium levels of fluorescence were determined by recording emission spectra of 6-MI (excitation at 340 nm) with an LS-55 spectrofluorometer (Perkin Elmer, Waltham, MA, USA) at 25 °C. The fluorescence at peak emission wavelength (420 nm) was used for data analysis and representation. Preassembled TECs were diluted at 50–100 nM into 500 μl of TB10D buffer, supplemented with 40 pM pyrophosphatase in a Quartz SUPRASIL Macro/Semi-micro Cell (Perkin Elmer; catalogue number B0631132) and the initial fluorescence was recorded. NTP substrates (5 μM) and RNAP inhibitors were then sequentially added into the cuvette under continuous mixing and incubated for 5 min before taking each reading. Time-resolved measurements were performed in an Applied Photophysics (Leatherhead, UK) SX.18MV stopped-flow instrument at 25 °C. The reaction was initiated by mixing 60 μl of 0.2 μM TEC with 60 μl of 400 μM NTP. Both solutions were prepared in TB10D buffer and, where indicated, supplemented with 0.4–250 μM CBR703. 6-MI fluorophore was excited at 340 nm and emitted light was collected through 400 nm longpass filters. At least three individual traces were averaged for each reported curve. Single-round pause assays TECs were formed for 15 min at 37 °C with 30 nM linear PCR-generated pIA171 template and 40 nM RNAP holoenzyme in 20 mM Tris-acetate, 20 mM Na-acetate, 2 mM Mg-acetate, 14 mM 2-mercaptoethanol, 0.1 mM EDTA and 4% glycerol, pH 7.9. To halt RNAP after the addition of A29, synthesis was initiated in the absence of UTP, with 150 μM ApU, 5 μM ATP and GTP, and 1 μM CTP supplemented with [α- 32 P]-CTP. For β′H777A enzyme, ATP and GTP were used at 50 μM and CTP at 10 μM to allow for efficient halted complex formation. Halted complexes were incubated with CBR703 (or dimethylsulphoxide) for 3 min at 37 °C. Transcription was restarted by addition of one-tenth volume of 100 μM GTP, 1.5 mM CTP, ATP and UTP, and 250 μg ml −1 rifapentin. Samples were removed at 7, 15, 30, 45, 60, 120, 180, 300 and 480 s and after a final 5 min incubation with 200 μM GTP (chase), and were quenched by addition of an equal volume of 10 M urea, 50 mM EDTA, 45 mM Tris-borate; pH 8.3, 0.1% bromophenol blue and 0.1% xylene cyanol. RNAs were separated on 8% denaturing polyacrylamide gels and quantified using a Typhoon FLA 9000 scanner (GE Healthcare), ImageQuant Software and Microsoft Excel. Each assay was performed in triplicate. Docking experiments The three-dimensional structures of CBR703, CBR9379 and CBR9393 were built in Discovery Studio 3.5 (Accelrys, San Diego, CA, USA) and optimized using Minimize Ligands protocol and CHARMM force field [46] . In CBR703 and CBR9379 benzene rings interconnected by N -hydroxyamidine, moiety were modelled in cis –configuration, whereas N -hydroxyamidine and carbamide (in CBR9379) moieties were modelled planar with non-rotable C-N and C-O bonds. In CBR9393, the bond between the benzene ring and α-nitrogen of piperazinylethylamino group was set non-rotable, whereas ternary nitrogen of piperazinyl moiety was protonated and positively charged during docking runs. RNAP fragment comprising amino-acid residues within 20 Å from the putative CBR-binding cavity ( Supplementary Data 4 ) was extracted from E. coli RNAP holoenzyme crystal structure (PDB 4IGC) [37] and prepared for docking using Prepare Protein protocol of Discovery Studio (for GOLD runs) and AutoDock tools [47] (for AutoDock Vina runs). GOLD 5.2 (refs 35 , 36 ) docking runs were performed using LIGSITE-binding cavity detection algorithm [48] and GoldScore scoring function. AutoDock Vina 1.1.2 docking runs were performed in 25 × 25 × 18 Å 3 search space centred at 130.9, 6.8, −6.7 Å (coordinate space of Supplementary Data 1–4 ) using default scoring function [34] . Data analyses Time-resolved nucleotide incorporation and translocation data were simultaneously fit to a three-step model using the numerical integration capabilities of KinTek Explorer software [49] (KinTek Corporation). The model postulated that the initial TEC16 slowly and reversibly interconverts between inactive and active states and, on the addition of the NTP substrate, undergoes an irreversible transition to TEC17, followed by irreversible translocation except for β′F773V and β′P750L RNAPs where translocation was modelled as a reversible process. Equilibrium titration data were fit to the dissociation equilibrium equations that accounted for changes in concentrations of all reactants on complex formation using Scientist 2.01 software (Micromath, Saint Louis, MO, USA). These models are described in detail in Supplementary Methods . How to cite this article: Malinen, A. M. et al . CBR antimicrobials alter coupling between the bridge helix and the β subunit in RNA polymerase. Nat. Commun. 5:3408 doi: 10.1038/ncomms4408 (2014).